Genomic landscape of paediatric adrenocortical tumours Paediatric adrenocortical carcinoma is a rare malignancy with poor prognosis. Here we analyse 37 adrenocortical tumours (ACTs) by whole-genome, whole-exome and/or transcriptome sequencing. Most cases (91%) show loss of heterozygosity (LOH) of chromosome 11p, with uniform selection against the maternal chromosome. IGF2 on chromosome 11p is overexpressed in 100% of the tumours. TP53 mutations and chromosome 17 LOH with selection against wild-type TP53 are observed in 28 ACTs (76%). Chromosomes 11p and 17 undergo copy-neutral LOH early during tumorigenesis, suggesting tumour-driver events. Additional genetic alterations include recurrent somatic mutations in ATRX and CTNNB1 and integration of human herpesvirus-6 in chromosome 11p. A dismal outcome is predicted by concomitant TP53 and ATRX mutations and associated genomic abnormalities, including massive structural variations and frequent background mutations. Collectively, these findings demonstrate the nature, timing and potential prognostic significance of key genetic alterations in paediatric ACT and outline a hypothetical model of paediatric adrenocortical tumorigenesis. Adrenocortical tumours (ACTs) are rare [1] . A good outcome, as with most paediatric embryonal tumours, requires early diagnosis and complete surgical resection. Children with locally advanced or metastatic disease have a very poor prognosis, even with surgery and intensive chemotherapy [2] . Childhood ACT is often associated with germline TP53 mutations (Li-Fraumeni syndrome) [3] or constitutional genetic and/or epigenetic alterations affecting chromosome 11p15 (Beckwith-Wiedemann syndrome, BWS) [4] . Both Li-Fraumeni syndrome and BWS have highly variable phenotypes, which include susceptibility to ACT and other embryonal malignancies [5] . The factors contributing to sporadic paediatric ACTs are unknown, although the similarity of these cases to those with a constitutional predisposition suggests a common mechanism of tumorigenesis [1] . ACT is uniquely amenable to molecular studies relevant to paediatric embryonal neoplasms in general. First, the marked clinical endocrine manifestations of ACT (for example, virilization and Cushing syndrome) allow access to tumour tissue at an early disease stage. Second, ACT shares the epidemiological and molecular features of embryonal tumours [5] . Finally, a cluster of ACTs arising from a founder TP53 mutation (R337H) in southern Brazil allows biologic, prognostic and therapeutic studies in a relatively large group of cases with a common predisposing factor [6] , [7] , [8] , [9] . Staging of paediatric ACT is based on tumour size and evidence of residual tumour after surgery [1] . Histopathologic classification criteria, which have been invaluable in distinguishing adenoma (benign) from carcinoma (malignant) in adult ACTs [10] , have a limited role in guiding therapeutic decisions in paediatric ACTs, the great majority of which are classified as carcinomas or histology of undetermined malignant potential [11] , [12] . To advance our understanding of the initiation and progression of paediatric ACT, we undertook a comprehensive genomic analysis of 37 representative cases, including 12 tumours associated with the germline TP53 -R337H mutation, using a combination of whole-genome sequencing (WGS), whole-exome sequencing (WES) and transcriptome profiling (RNA-seq). 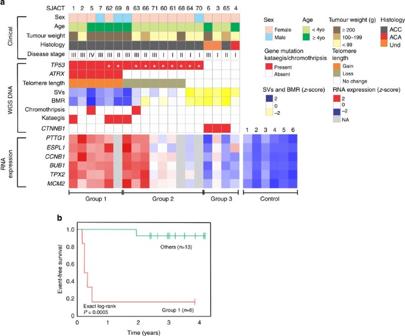Figure 1: Association between molecular and clinicopathological features of paediatric adrenocortical tumours. (a) Upper panel: clinicopathological features of 19 patients in the WGS cohort. Centre panel: genetic alterations, including mutational status ofTP53(R337H identified by asterisk),ATRXandCTNNB1;telomere length; number of SVs; BMR; chromothripsis and kataegis. Und: undetermined malignancy. Lower panel: RNA expression of selected genes involved in chromosomal segregation and cell cycle control. Three distinct tumour groups (labelled below) emerged from this analysis. Control: normal adrenocortical tissue. (b) Kaplan–Meier probability of event-free survival (exact log-rank test) of paediatric ACT patients in group 1 versus others. Clinical data The clinical and biological characteristics of the 37 newly diagnosed ACT cases studied by WGS and WES are summarized in Supplementary Table 1a,b . The median age of the 25 girls and 12 boys at diagnosis was 53.5 months (range, 9.7–184.7 months). Tumours were sporadic ( n =10) or associated with constitutional cancer predisposition conditions (Brazilian founder TP53 -R337H ( n =12); other types of germline TP53 mutations ( n =13) and BWS ( n =2)) and included 29 carcinomas, 3 adenomas and 5 tumours of undetermined malignant potential. These cases were selected on the basis of availability of paired tumor and germline samples and isolation of high-quality tumour DNA. Although treatment was not uniform, it generally adhered to the Children’s Oncology Group (COG) ARAR0332 protocol [1] , consisting of surgery alone for stage I and II disease, and surgery followed by intensive chemotherapy (cisplatin, doxorubicin, etoposide and mitotane) for advanced-stage (III and IV) disease. At a median follow-up of 38 months, 11 of 35 (31%) patients had experienced an adverse event (relapse or death). Five of these eleven had died of progressive disease at the time of this report, and six remained alive in second complete remission. Two patients were lost to follow-up. Clinical data from 34 additional ACT patients studied as an independent comparison group (‘convenience cohort’) is included in Supplementary Table 1c . 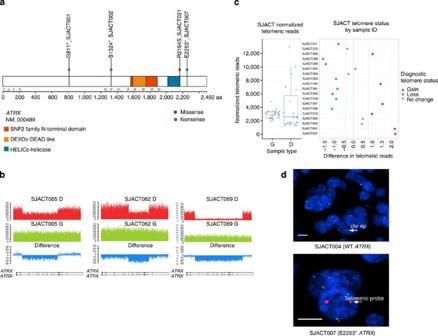Figure 2: SomaticATRXmutations and telomere analysis of paediatric adrenocortical tumours. (a) Distribution of nonsilent single-nucleotide variations inATRX(blue dots: nonsense mutations; red dot: missense mutation). (b) Wiggle plots showing internal deletion of multiple exons in theATRXgene in SJACT005, SJACT062 and SJACT069 (diagnostic tumour [D] and germline [G] samples). (c) Relative telomere length determined by WGS in paediatric ACTs versus matched germline samples. (d) Images of tumour samples hybridized with the telomeric FISH (red) and chromosome 4p (green) probes and stained with DAPI to visualize the nucleus (blue). High-magnification views show the large, ultrabright signal inATRX-mutant adrenocortical tumour cells (SJACT007). Scale bars, 1 μm. Genome and transcriptome analyses Primary ACTs and matched peripheral blood DNA were analysed by WGS ( n =19) at an average 41.9X coverage ( Supplementary Table 2a ) or by WES ( n =18) at an average 84.8X coverage ( Supplementary Table 2b ; Pediatric Cancer Genome Project, http://pcgpexplore.org/ ). All genetic lesions, including single-nucleotide variations (SNV), small insertions/deletions (indels) and structural variations (SVs), were experimentally validated ( Supplementary Fig. 1 ). 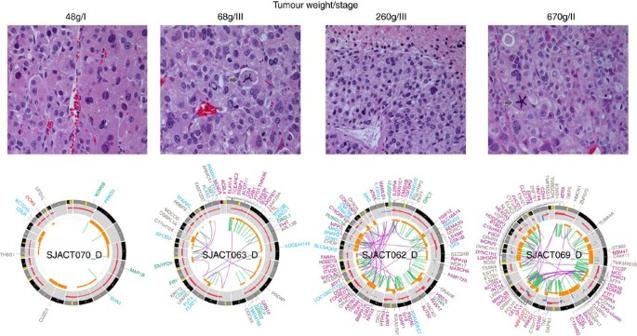Figure 3: Histopathological and genomic features ofTP53-R337H-associated ACTs. All tumours had a high mitotic rate (>5 per 50 high-power fields, H&E, × 400). Histology showed a vague nested and trabecular pattern with occasional unpatterned cellular sheets of variable size. Three cases (SJACT063, SJACT062 and SJACT069) had a high nuclear grade and marked cellular pleomorphism. SJACT070 showed occasional enlarged hyperchromatic nuclei with one or more prominent nucleoli. Necrotic cells and atypical mitotic figures (arrow) are identified in SJACT63 and SJACT69. Accumulation of genomic alterations illustrated by the Circos plots (bottom panels) paralleled an increase in tumour weight and correlated with a more aggressive tumour phenotype (Group 1 versus Group 2). Note: labels for gene-disrupting SVs (SJACT063 and SJACT062) and noncoding mutations (SJACT069) were removed from the Circos plots. In the WGS samples, the median number of nonsilent point mutations was 5 (range, 1–97), the median background mutation rate (BMR) was 3.78 × 10 −7 (range, 5.01 × 10 −8 –2.40 × 10 −6 ) and the median number of SVs per case was 61 (range, 0–812; Supplementary Table 3a–d ). Transcriptome profiles of normal adrenocortical tissue ( n =6) and ACT samples from the WGS cohort ( n =16) were analysed using RNA sequencing (RNA-seq; Supplementary Table 2c ). TP53 mutations Germline TP53 mutations were present in 25 of the 37 patients (68%) in the combined WGS and WES cohorts, 12 of which were the Brazilian founder R337H mutation ( Fig. 1a and Supplementary Fig. 3a ). Somatic mutations (R175H, R273C and a homozygous deletion of ~200 kb of chromosome 17 encompassing TP53 ) were also identified in 3 of the 12 ACTs associated with wild-type germline TP53 ( Supplementary Fig. 3a,b ). Figure 1: Association between molecular and clinicopathological features of paediatric adrenocortical tumours. ( a ) Upper panel: clinicopathological features of 19 patients in the WGS cohort. Centre panel: genetic alterations, including mutational status of TP53 (R337H identified by asterisk), ATRX and CTNNB1; telomere length; number of SVs; BMR; chromothripsis and kataegis. Und: undetermined malignancy. Lower panel: RNA expression of selected genes involved in chromosomal segregation and cell cycle control. Three distinct tumour groups (labelled below) emerged from this analysis. Control: normal adrenocortical tissue. ( b ) Kaplan–Meier probability of event-free survival (exact log-rank test) of paediatric ACT patients in group 1 versus others. Full size image Sanger sequencing identified germline TP53 mutations in 11 of the 34 cases (32%) in the independent comparison cohort ( Supplementary Table 1c ). Of the 23 ACTs in this group associated with germline wild-type TP53 , three tumours acquired a TP53 mutation (c.134_135 insT, E180K and R273H; Supplementary Fig. 4a ). Somatic ATRX mutations ATRX encodes a helicase that functions in chromatin remodelling and telomere structural maintenance, and it cooperates with DAXX to incorporate the histone variant H3.3 into chromatin [13] . ATRX somatic nonsense mutations and SVs deleting multiple exons were identified by WGS in 6 of the 19 ACTs (32%), all of which were associated with germline TP53 mutations ( Fig. 1a and 2a,b ). An ATRX somatic missense mutation (R2164S) was also identified by WES in the case with somatic homozygous deletion of TP53 ( Fig. 2a and Supplementary Fig. 3b ). No mutations were detected in the coding region of DAXX or TERT by WGS or WES. Furthermore, no mutations were identified in the TERT core promoter by targeted Sanger sequencing. Although broad regional amplification encompassing the TERT locus was observed in 13 of the 19 WGS cases (68%), no TERT expression was detected with RNA-seq. Figure 2: Somatic ATRX mutations and telomere analysis of paediatric adrenocortical tumours. ( a ) Distribution of nonsilent single-nucleotide variations in ATRX (blue dots: nonsense mutations; red dot: missense mutation). ( b ) Wiggle plots showing internal deletion of multiple exons in the ATRX gene in SJACT005, SJACT062 and SJACT069 (diagnostic tumour [D] and germline [G] samples). ( c ) Relative telomere length determined by WGS in paediatric ACTs versus matched germline samples. ( d ) Images of tumour samples hybridized with the telomeric FISH (red) and chromosome 4p (green) probes and stained with DAPI to visualize the nucleus (blue). High-magnification views show the large, ultrabright signal in ATRX -mutant adrenocortical tumour cells (SJACT007). Scale bars, 1 μm. Full size image WGS-based telomere length analysis showed an increase in telomeric DNA in all six tumours with ATRX mutations, but not in tumours with wild-type ATRX ( P =3.7 × 10 −5 , Fisher’s exact test; Fig. 2c ). Telomere fluorescence in situ hybridization (FISH) analysis of 22 available formalin-fixed, paraffin-embedded tumour specimens revealed large, ultrabright telomere foci ( Fig. 2d ) in cases harbouring ATRX mutations ( n =5), suggesting the activation of an alternative lengthening of telomere mechanism. Telomere foci were also observed in the SJACT023 tumour, although WES did not detect an ATRX mutation. Somatic β-catenin mutations Somatic β -catenin ( CTNNB1 ) mutations were identified in 3 of the 37 (8%) tumours analysed in the combined WGS and WES cohorts ( Fig. 1a and Supplementary Fig. 5 ). Targeted Sanger sequencing of CTNNB1 exon 3 revealed 10 additional somatic mutations in 34 paediatric ACTs in the independent comparison cohort ( Supplementary Fig. 4b ). Overall, CTNNB1 mutations ( n =13) were detected only in tumours with wild-type germline TP53 ( n =35) and not in those with constitutional TP53 mutations ( n =36; P =2.5 × 10 −5 , Fisher’s exact test). However, three tumours with somatic CTNNB1 mutations had also acquired a TP53 mutation (IPACTR001, IPACTR013 and IPACTR019; Supplementary Fig. 4b and Supplementary Table 1c ). Genomic classification of ACT WGS defined three groups of paediatric ACT based on the mutational status of TP53 and ATRX : Group 1 germline TP53 and somatic ATRX mutations ( n =6); Group 2 germline TP53 mutations and no ATRX mutation ( n =9); and Group 3 both wild-type TP53 and ATRX ( n =4; Fig. 1a ). Group 1 cases had significantly greater tumour weight ( P =0.007, Mann–Whitney test), were significantly more likely to have stage 3 or 4 disease ( P =0.020, Kendall test) and had poorer event-free survival than Groups 2 and 3 ( P =5.0 × 10 −5 , exact log-rank test; Fig. 1a,b ). Group 1 ACTs also had a significantly larger number of SVs ( P =0.021, Mann–Whitney test) and higher BMR ( P =0.015, Mann–Whitney test; Supplementary Fig. 3c ). In addition, these tumours showed significantly higher expression of genes associated with chromosome instability and deregulation of cell cycle control ( PTTG1 , P =0.019; ESPL1 , P =0.015; CCNB1 , P =0.018; BUB1 , P =0.023; TPX2 , P =0.032; and MCM2 , P =0.040, t -test; Fig. 1a ). Although all cases in Group 2 carried germline TP53 mutations (eight of nine cases had the founder R337H mutation and were diagnosed in southern Brazil), they displayed variable clinical findings. Group 2 patients with the R337H mutation were young (median age, 30 months), exhibited signs of virilization and had relatively small tumours (median tumour weight 68 versus 585 g in Group 1 ( P <0.006, Wilcoxon rank sum test)). These tumours showed variable numbers of SVs and BMR, and variable expression of selected target genes ( Fig. 1 and Supplementary Fig. 3c ). A distinguishing feature of this group is the lack of ATRX mutations and the shortening of telomeres as compared with Group 1. Group 3 tumours showed a relatively small number of SVs and a low BMR, and gene expression of those selected genes was similar to that in normal adrenocortical tissue, consistent with their more favourable outcome ( Fig. 1 and Supplementary Fig. 3c ). WGS did not reveal any specific genetic alterations that distinguished ACTs harbouring the founder TP53 -R337H from tumours with other TP53 mutations. However, R337H tumours that had acquired an ATRX mutation (cases SJACT062 and SJACT069) clustered in Group 1 and exhibited an aggressive phenotype ( Figs 1 and 3 ). The remaining eight R337H cases showed variable molecular profiles and disease stage ( Fig. 1 and Supplementary Fig. 2 ). Figure 3 illustrates the relationship among histopathological features, tumour weight, stage and complexity of genomic abnormalities for four cases with the same predisposing TP53 -R337H germline mutation. Figure 3: Histopathological and genomic features of TP53 -R337H-associated ACTs. All tumours had a high mitotic rate (>5 per 50 high-power fields, H&E, × 400). Histology showed a vague nested and trabecular pattern with occasional unpatterned cellular sheets of variable size. Three cases (SJACT063, SJACT062 and SJACT069) had a high nuclear grade and marked cellular pleomorphism. SJACT070 showed occasional enlarged hyperchromatic nuclei with one or more prominent nucleoli. Necrotic cells and atypical mitotic figures (arrow) are identified in SJACT63 and SJACT69. Accumulation of genomic alterations illustrated by the Circos plots (bottom panels) paralleled an increase in tumour weight and correlated with a more aggressive tumour phenotype (Group 1 versus Group 2). Note: labels for gene-disrupting SVs (SJACT063 and SJACT062) and noncoding mutations (SJACT069) were removed from the Circos plots. Full size image Loss of heterozygosity of chromosomes 11 and 17 Chromosome 17 loss of heterozygosity (LOH) was observed in 28 of the 37 ACTs (76%) by WGS and WES. All tumours with germline ( n =25) and somatic ( n =3) TP53 mutations underwent LOH with selection against the wild-type allele ( Supplementary Fig. 2 ). More specifically, WGS demonstrated copy-neutral LOH (cn-LOH) of the entire chromosome 17 in all tumours associated with germline TP53 mutations ( n =15), as well as in two (SJACT003 and SJATC004) of the four cases with wild-type TP53 ( Supplementary Fig. 2 ). Chromosome 11p LOH was also identified in 32 of the 35 ACTs (91%). Two BWS patients (SJACT009 and SJACT065) with germline 11p homozygosity, indicative of uniparental disomy, were excluded from the analysis as LOH could not be assessed ( Supplementary Fig. 2 and Fig. 4a ). Furthermore, cn-LOH of chromosome 11p was demonstrated by WGS in 14 of the 18 informative ACTs ( Supplementary Fig. 2 ). Microsatellite marker analysis of an additional 22 paediatric ACT cases from our independent comparison cohort revealed chromosome 11p LOH in 20 tumours (95%, as IPACTR004 was excluded due to uniparental disomy; Supplementary Fig. 4c ). Remarkably, 100% of the cases from the combined cohorts that underwent chromosome 11p15 LOH and had available parental DNA ( n =23) selectively retained the paternal chromosome ( P =2.4 × 10 −7 , sign test; Fig. 4a and Supplementary Fig. 4c ). 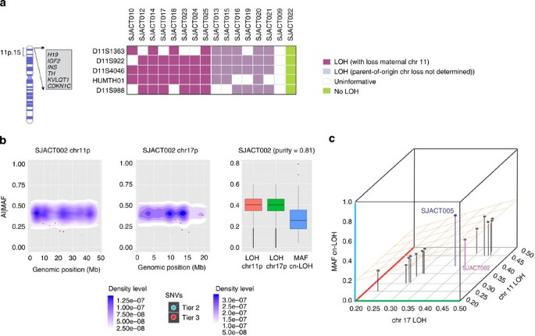Figure 4: Characterization and timing of chromosome 11 and 17 LOH in paediatric ACT. (a) Microsatellite analysis of chromosome 11p15 in the WES cohort. All cases with available parental DNA demonstrated selective loss of maternal chromosome 11p15 (n=8, purple). (b) Temporal order of chromosome 11p and 17p cn-LOH and accumulation of SNVs in SJACT002. Scatter plots show MAFs of somatic SNVs and their genomic positions (individual dots) combined with two-dimensional (2D) density plots of AI values of germline heterozygous SNPs in cn-LOH regions of chromosomes 11p (left) and 17p (centre). At right, AI values in cn-LOH regions of chromosomes 11p and 17p were compared with the MAF distribution of somatic SNVs in genome-wide cn-LOH regions. (c) A three-dimensional (3D) scatter plot summarizes the temporal order of cn-LOH of chromosomes 11p and 17p and somatic SNV accumulation in paediatric ACTs. Shown are the median AI values for the chromosome 11p cn-LOH region, the median AI values for the chromosome 17p cn-LOH region and the median MAF of SNVs in genome-wide cn-LOH regions of 14 cases; SJACT002 and SJACT005 are labelled. See alsoSupplementary Fig. 7b. Figure 4: Characterization and timing of chromosome 11 and 17 LOH in paediatric ACT. ( a ) Microsatellite analysis of chromosome 11p15 in the WES cohort. All cases with available parental DNA demonstrated selective loss of maternal chromosome 11p15 ( n =8, purple). ( b ) Temporal order of chromosome 11p and 17p cn-LOH and accumulation of SNVs in SJACT002. Scatter plots show MAFs of somatic SNVs and their genomic positions (individual dots) combined with two-dimensional (2D) density plots of AI values of germline heterozygous SNPs in cn-LOH regions of chromosomes 11p (left) and 17p (centre). At right, AI values in cn-LOH regions of chromosomes 11p and 17p were compared with the MAF distribution of somatic SNVs in genome-wide cn-LOH regions. ( c ) A three-dimensional (3D) scatter plot summarizes the temporal order of cn-LOH of chromosomes 11p and 17p and somatic SNV accumulation in paediatric ACTs. Shown are the median AI values for the chromosome 11p cn-LOH region, the median AI values for the chromosome 17p cn-LOH region and the median MAF of SNVs in genome-wide cn-LOH regions of 14 cases; SJACT002 and SJACT005 are labelled. See also Supplementary Fig. 7b . Full size image Human chromosome 11p15 contains a large cluster of imprinted genes, including IGF2 , CDKN1C , KCNQ1 and H19 . IGF2 is a paternally expressed fetal growth factor, whereas the cell cycle inhibitor CDKN1 C (p57), potassium channel protein KCNQ1 and the noncoding H19 transcripts are expressed from the maternal allele. Expression of genes localized at 11p15 (chr11:1704500–3658789) was analysed with transcriptome profiling. RNA-seq confirmed greater expression of IGF2 in all tumours in the WGS cohort compared with normal adrenocortical tissue ( P =2.987 × 10 −7 , t -test; Supplementary Fig. 6 ). Expression of KCNQ1 , CDKN1C and H19 was low in most cases, consistent with loss of the maternal chromosome 11p. SJACT006, which retained both parental copies of chromosome 11, also displayed elevated IGF2 expression and deregulation of maternally expressed genes, suggesting a loss of imprinting control at this locus ( Supplementary Fig. 6 ). Timing of cn-LOH of chromosomes 11 and 17 To infer the temporal order of somatic SNV acquisition and cn-LOH in chromosomes 11 and 17, we compared the mutant allele fractions (MAFs) of SNVs in cn-LOH regions to allelic imbalance (AI) values, which express the different MAFs (germline heterozygous single-nucleotide polymorphisms (SNPs)) in tumour versus germline samples ( Fig. 4b,c and Supplementary Fig. 7 ). A cn-LOH event in the tumour cells will lead to an expected AI value of 0.5. Similarly, somatic SNVs acquired before cn-LOH would result in either a homozygous reference allele (R) or a homozygous mutant (M) allele, while SNVs accumulated after cn-LOH would remain heterozygous in the absence of a second hit ( Supplementary Fig. 7a ). Our analysis of 14 informative WGS samples demonstrated that most SNVs in chromosomes 11p and 17p were acquired after cn-LOH, although SJACT005 underwent cn-LOH during SNV accumulation ( Fig. 4b,c and Supplementary Fig. 7b ). These findings indicate that cn-LOH of chromosomes 11p and 17p occurs early in adrenocortical tumorigenesis and precedes the accumulation of SNVs in these regions. Chromosomal integration of human herpesvirus-6 Human herpesvirus-6 (HHV6) was detected by WGS in the germline and tumour DNA of SJACT004 ( Fig. 5a ) and by Sanger sequencing in SJACT017. FISH analysis confirmed the site of chromosomal integration of HHV6 as the telomeric region of 11p in both cases ( Fig. 5b ). PCR analysis demonstrated paternal transmission of chromosomally integrated HHV6 in SJACT017 ( Fig. 5c ). Microsatellite marker analysis and WGS confirmed chromosome 11 LOH with retention of integrated HHV6 in both cases ( Supplementary Figs 2 and 4c and Fig. 4a ). Genomic and transcriptome analyses of SJACT004 identified few somatic SNVs and SVs, but showed elevated IGF2 expression ( Supplementary Figs 2 and 6 ). Both ACTs were small, stage 1 tumours and with good prognosis ( Supplementary Table 1a,b ). 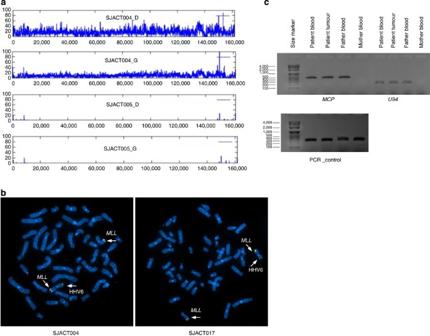Figure 5: Chromosomal integration of human herpesvirus-6 in paediatric ACT. (a) Coverage plot for cases SJACT004 and SJACT005 showing diagnostic tumour (D) and germline (G) samples reveals integration of the full-length HHV6 genome in SJACT004. The HHV6 genome is duplicated in the tumour sample as a consequence of cn-LOH. (b) FISH of metaphase chromosomes from peripheral blood confirmed HHV6 integration at 11p in both cases. TheMLLprobe (chromosome 11q23) was used as control (left, SJACT004; right, SJACT017). (c) HHV6MCP(major capsid protein) andU94were amplified with PCR from SJACT017 (germline and tumour) and parental DNA demonstrating paternal vertical transmission of integrated HHV6. Exon 6 of theTP53gene was amplified as DNA quality control. Figure 5: Chromosomal integration of human herpesvirus-6 in paediatric ACT. ( a ) Coverage plot for cases SJACT004 and SJACT005 showing diagnostic tumour (D) and germline (G) samples reveals integration of the full-length HHV6 genome in SJACT004. The HHV6 genome is duplicated in the tumour sample as a consequence of cn-LOH. ( b ) FISH of metaphase chromosomes from peripheral blood confirmed HHV6 integration at 11p in both cases. The MLL probe (chromosome 11q23) was used as control (left, SJACT004; right, SJACT017). ( c ) HHV6 MCP (major capsid protein) and U94 were amplified with PCR from SJACT017 (germline and tumour) and parental DNA demonstrating paternal vertical transmission of integrated HHV6. Exon 6 of the TP53 gene was amplified as DNA quality control. Full size image Other genetic events Chromosomal copy number alterations (CNAs) were also assessed by a modified version of GISTIC (genomic identification of significant targets in cancer). Deletion of chromosome 4q34 was observed in 11 of the 19 tumours (58%; Supplementary Fig. 8a,b ). The most commonly deleted region overlapped a 5-Mb area encompassing LINC00290 (long intergenic nonprotein-coding RNA 290) [14] . Chromosomal copy number gains were widespread, with 9q being over-represented and amplified in 16 of the 19 WGS ACTs, similar to previously reported findings ( Supplementary Fig. 8a,c ) [14] . Chromosome shattering consistent with chromothripsis [15] ( Supplementary Fig. 9 ) and patterns of localized hypermutation (kataegis [16] ; Supplementary Fig. 10 ) were observed in late-stage tumours ( Fig. 1a ). Structural variants resulting in the expression of fusion genes were infrequent and nonrecurrent ( Supplementary Table 4 ). Our genomic findings define cn-LOH of chromosome 11p, with selection against the maternal chromosome and consequent IGF2 overexpression, as an early event and a hallmark of paediatric adrenocortical tumorigenesis. Although paediatric ACT is strongly associated with germline TP53 mutations [17] , [18] , [19] (60–70% of children with ACT [3] ), only 4–6% of carriers develop ACTs [1] , suggesting the involvement of cooperating genetic alterations. We propose that germline TP53 mutations may contribute to adrenocortical tumorigenesis by promoting chromosomal instability [20] , [21] . In this setting, aneuploid adrenocortical cells that experience chromosome 11p LOH and deregulation of imprinted genes on 11p15 may be selected and expanded via constitutive overexpression of IGF2 , which encodes a potent mitogen and fetal growth-promoting protein [22] , [23] . This mechanism is consistent with chromosome 11p abnormalities and IGF2 overexpression in all cases of ACT with germline TP53 mutations. Clones that undergo chromosome 17 LOH and lose wild-type TP53 become more unstable, accumulate additional SNVs and are selected for further expansion. In support of this hypothesis, our temporal studies place cn-LOH of chromosomes 11p and 17 during early tumorigenesis, before the acquisition of widespread genomic alterations. Our WGS study included 10 Brazilian cases with the founder TP53 -R337H mutation, which could influence the resulting genomic landscape findings. TP53 -R337H is a missense mutation that is partially functional [6] , [24] ; hence, we expected that genomic changes could be different from those with nonfunctional mutations. Our genomic studies showed that some cases with the R337H mutation had secondary genetic events that were similar to those seen with other types of TP53 mutations, such as concomitant cn-LOH of chromosomes 11 and 17p early during tumorigenesis, as well as the deregulation of IGF2 expression and acquired ATRX mutations. These findings are consistent with those from high-density SNP analysis that demonstrated that the pattern of gains and losses is similar in paediatric ACTs with R337H and other TP53 mutations [14] . However, other cases with R337H mutations had much simpler genomes similar to those with wild-type TP53 . It is possible that secondary genomic changes increase with time from tumour initiation to diagnosis. Alternatively, other genetic constitutional or acquired changes account for the observed heterogeneity observed in cases with the R337H mutations. Further studies will be required to examine these possibilities. LOH of chromosome 11p15 and genomic imprinting abnormalities within this region that lead to constitutive IGF2 expression are features of many other paediatric tumours, including rhabdomyosarcoma [25] , Wilms tumour [26] and hepatoblastoma [27] . Similarly, adult adrenocortical carcinomas, but not adenomas, show genomic imprinting abnormalities at chromosome 11p15 (refs 28 , 29 ). However, transgenic mouse models demonstrate that IGF2 overexpression is not by itself sufficient to promote adrenocortical tumorigenesis [30] but must cooperate with other genetic alterations, such as activation of β-catenin [31] . Consistent with these findings, CTNNB1 -activating mutations were relatively frequent in our cohort, particularly in cases with germline wild-type TP53 . Assié et al . [29] recently reported the characterization of 45 adult adrenocortical carcinomas (ACCs) using an integrated genomic analysis approach. A comparison of our findings to this published study highlights similarities and differences in the genetic changes that occur in paediatric and adult ACTs ( Supplementary Table 5 ). Remarkably, 11p15 LOH involving the IGF2 locus was observed in both paediatric ACT (91%) and adult ACC (82%), underscoring the critical role of deregulated IGF2 expression in adrenal cortex tumorigenesis. Aneuploidy with widespread chromosomal gains (for example, chromosome 19) and deletions (for example, 4q34.3) was also observed in both paediatric and adult cases. However, amplification of chromosome 9q, a region that includes NOTCH1 and NR5A1 ( Steroidogenic Factor-1 ), occurred in 90% of paediatric ACTs ( Supplementary Fig. 8a,c ), but not in adult ACC [29] . Activating mutations in CTNNB1 were common to both paediatric and adult ACT, but additional mutations within the Wnt/β-catenin signalling pathway, in particular ZNRF3 , were only observed in adult tumours. Germline TP53 mutations were predominantly associated with paediatric ACT, whereas somatic TP53 mutations were relatively infrequent in both groups. The alternative lengthening of telomere phenotype was associated with DAXX or ATRX mutations in adult tumours, but exclusively with ATRX mutations in paediatric cases. Amplification of TERT was common in both groups, but no TERT mutations were detected in the paediatric cases, consistent with the absence of TERT expression. A lack of strong prognostic indicators has limited progress in the management of childhood ACT. Overall event-free survival is only ~50%, and patients with advanced-stage disease have very poor overall survival [1] , [2] . Unlike studies of other paediatric embryonal tumours [32] , [33] , [34] , histopathological examination [11] and molecular findings [35] in paediatric ACT has not produced relevant prognostic categories or novel treatment approaches. Tumour weight, volume and surgical resectability form the basis of the current COG disease-stage classification [1] . However, this system needs improvement, as many patients experience relapse despite small, completely excised tumours, while others are cured despite histological findings suggestive of carcinoma [36] . Our genomic analysis opens opportunities to improve the current tumour size-histology-disease stage prognostic scheme for paediatric ACT [1] , [2] . Notably, tumours with both germline TP53 and somatic ATRX mutations (Group 1) were significantly associated with high tumour weight, advanced disease (COG stage III/IV) and poor event-free survival. SJACT069 (R337H) exemplifies such a case; it was staged as limited disease (COG stage II) and initially managed with surgery alone, but later metastasized to the lungs. Moreover, five of six patients in Group 1 had adverse events (relapse or death), consistent with the genomic findings indicative of an aggressive phenotype. Cases with germline TP53 mutations and wild-type ATRX (Group 2) are clinically and molecularly heterogeneous. Although all cases in this group carried TP53 mutations (eight of the nine cases harbour the founder R337H), they had fewer genomic abnormalities, smaller tumours and generally much better clinical outcome than cases in Group 1. It is not surprising that patients in southern Brazil with the R337H mutation were diagnosed earlier, as paediatricians of that region are familiar with the first signs of ACT and promptly refer these children for treatment. However, three patients (one with the TP53 G245C and two with the Brazilian R337H mutation) overexpressed genes associated with chromosome instability and cell cycle control ( Fig. 1a ; Supplementary Table 1 ). The two cases with R337H required chemotherapy because of advanced-stage disease in one and tumour rupture in the other. The patient with the G245C, a child more than 10 years of age at diagnosis of ACT, had delayed diagnosis of a very large tumour in the absence of endocrine signs (a ‘nonfunctional’ tumour). This child was treated with surgery followed by chemotherapy, but eventually died of relapsed disease. These observations suggest that paediatric TP53 -associated tumours arise from a simpler genomic background (adenoma or undetermined malignant potential) and progress to acquire complex and unstable genomic aberrations (carcinoma). The results of newborn screening for the TP53 mutation in Brazil and surveillance of carriers for early signs of ACT [9] are consistent with this concept [37] . Finally, ACTs with wild-type TP53 exhibit relatively simple genomes and, despite their large size in some cases, patients generally have a good outcome. Because of the small number of these cases, additional genomic studies will be needed to clarify the role of molecular changes in this subset of patients. In two of our cases (SJACT004 and SJACT017), HHV6 was selectively integrated into the telomeric region of chromosome 11p. HHV6 is known to integrate into the genome at a low frequency (~1%), preferring the telomeric regions of chromosomes 9q, 11p, 17p and 19q (refs 38 , 39 ). A recent report documented the role of integrated HHV6 in disrupting telomeres, leading to selective aneuploidy [40] . Whether chromosomal integration of HHV6 facilitates 11p cn-LOH and deregulation of imprinting at the 11p15 locus, leading to IGF2 overexpression, remains to be determined. In summary, our study identified key genetic alterations and their temporal relationships in paediatric adrenocortical tumorigenesis. The genomic complexity of childhood ACTs, particularly those with both germline TP53 and acquired ATRX mutations, may explain the failure of standard chemotherapy, underscoring the importance of early diagnosis and improved prognostic classification. Patients and samples Written informed consent was obtained from parents or legal guardians for inclusion in the St Jude Children’s Research Hospital (St Jude) International Pediatric Adrenocortical Tumor Registry (IPACTR; http://clinicaltrials.gov/show/NCT00700414 ) or for participation in COG ARAR0332 protocol ( http://clinicaltrials.gov/show/NCT00304070 ). IPACTR registers childhood cases of ACT worldwide. COG studies enroll patients from the United States, Canada and southern Brazil, where 90% of cases carry the founder TP53 -R337H mutation. Diagnosis was made on the basis of the gross and histologic appearance of tissue obtained at surgery. The diagnosis of ACT was centrally reviewed and confirmed. Tumours were further classified as adenoma (benign), carcinoma (malignant) or having histology of undetermined malignant potential. No attempt was made to obtain individual tumour scores. Samples for WGS ( n =19) and WES ( n =18) included matched peripheral blood and primary tumour tissue from 26 IPACTR patients and 11 COG patients. An additional group of 34 IPACTR patients with matched primary tumour and blood samples, and blood-derived DNA from 23 sets of parents, were included for analysis of chromosome 11p LOH, TP53 and CTNNB1 mutation. Six samples of normal adrenocortical tissue obtained during nephrectomy for Wilms tumour were used as controls in gene expression studies as well 16 tumour samples studied in the WGS cohort. All tumour samples underwent estimation of the purity-adjusted MAF, tumour purity and tumour heterogeneity and quantitative analysis of chromothripsis [41] . This study was approved by the St Jude Institutional Review Board and by the Cancer Therapy Evaluation Program of the National Cancer Institute (ARAR12B1). Tumour purity estimations For germline heterogeneous SNPs, LOH measures the absolute difference between the MAF in tumour and that in germline sample (0.5). LOH is the result of copy number alterations and/or cn-LOH in tumour cells. Compared with copy number gains (a single copy gain in 100% tumour results in a LOH value of 0.167), regions with copy number loss showed stronger LOH (a single copy loss in 100% tumour result in a LOH value of 0.5). Consequently, we used LOH signals in copy neutral or heterozygous copy number loss regions (CNA value between [−1, 0]) to estimate tumour purity for all WGS samples. Briefly, a single copy loss in x % tumour cells resulted in an estimated CNA value of and a LOH value of . Assuming that the remaining LOH signal came from cn-LOH (cn-LOH in x % tumour cell resulted in a LOH value of ), the tumour content in a region could be estimated as the sum of the fraction with copy number loss and the fraction with cn-LOH by: . Using tumour content estimates from various regions within the genome, we performed an unsupervised clustering analysis using the mclust package (version 3.4.8) in R (version 2.11.1). The tumour purity of the sample was defined as the highest cluster centre value among all clusters. Purity-adjusted MAF estimation MAF for validated SNVs was estimated as using deep sequencing data. Tumour heterogeneity estimation We used all validated autosomal SNVs satisfying the following criteria in heterogeneity analysis: 1 In copy neutral region (Log2ration between (−0.1, 0.1) in CNV analysis). 2 Not in regions with LOH (LOH value <0.1). 3 With MAF >0.05 or mutant allele count >2. We drew the kernel density estimate plot for MAFs of the qualifying SNVs using the density function in the stat package in R. We also estimated the number of significant peaks and the relative MAF component for each peak (peaks with less than five SNVs, peaks with less than 1% SNVs and peaks with excessive variance were ignored). A sample with heterogeneity shows density peaks at a MAF smaller than 0.5 (the expected MAF assuming heterogeneous SNVs). Kataegis analysis Kataegis analysis was performed on all validated Tier1–3 SNVs and SV breakpoints for each sample. The intermutation distance for a SNV was calculated as the distance to its nearest neighbour. For each SNV, its distance to the nearest validated SV breakpoint was also calculated. We defined microclusters of kataegis as clusters that contain at least five consecutive SNVs with intervariant distance less than 10 kb. Mutant allele frequency (MAF) was estimated for SNVs with at least 20 × coverage in tumour BAMs based on deep sequencing of custom capture validation. Whole-genome sequencing WGS was performed as previously described [42] , [43] . WGS mapping, coverage, quality assessment, SNV, indel detection, tier annotation for SNVs, prediction of deleterious effects of missense mutations and identification of LOH have been described previously [42] . SVs were analysed by using the CREST software and were being annotated as previously described [42] , [44] . The reference human genome assembly NCBI Build 37 was used for mapping samples. CNAs were identified by comparing read depth in tumour versus matched normal samples and using a novel algorithm, CONSERTING (COpy Number SEgmentation by Regression Tree In Next-Gen sequencing). SNVs were classified according to the following three tiers, as previously described [42] . Tier1: Coding synonymous, nonsynonymous and splice-site variants and noncoding RNA variants. Tier 2: Conserved variants (cutoff conservation score ≥500, based on either the phastConsElements28way table or the phastConsElements17way table from the UCSC genome browser ( http://genome.ucsc.edu/ ) and variants in regulatory regions annotated by UCSC annotation (regulatory annotations included targetScanS, ORegAnno, tfbsConsSites, vistaEnhancers,eponine, firstEF, L1 TAF1 Valid, Poly(A), switchDbTss, encodeUViennaRnaz, laminB1 and cpgIslandExt)). Tier 3: Variants in nonrepeat masked regions. Tier 4: All other SNVs. Exome sequencing For exome sequencing, DNA libraries were prepared from 1 μg of WGA DNA from matched samples by using the Illumina TruSeq DNA library prep kit according to the manufacturer’s protocol. The quality of library construction was assessed on an Agilent Bioanalyzer. Germline and diagnostic library samples were independently pooled for exome capture by using the Illumina TruSeq Exome Enrichment kit as instructed by the manufacturer. Captured libraries were then clustered on the Illumina c-bot and sequenced on an Illumina HiSeq 2000 platform by conducting 100 base pair-end-multiplexed reads at an equivalent of three samples per lane. Sequence validation To enrich regions containing putative sequence alterations, genomic coordinates of the WGS targets were used to order Nimbelgen Seqcap EZ solution bait sets (Roche). Library construction and target enrichment were performed as per the manufacturer’s instructions, using repli-G (Qiagen) WGA DNA. Enriched targets were sequenced on the Illumina platform by paired-end 100-cycle sequencing. The resulting data were converted to FASTQ files by using the CASAVA 1.8.2 (Illumina) programme and were mapped with a Burrows-Wheeler Aligner before pipeline analysis. Putative SNVs and indels from exon sequencing were validated by next-generation amplicon sequencing. Briefly, primers were designed for genomic regions (hg19) flanking the detected SNV but no nearer than 100 base pairs. PCR was performed by using 20–30 ng of WGA DNA from each sample. DNA from diagnostic tumour samples and matched germline samples was used for each primer set to confirm the presence of the SNV/indel in the diagnostic sample. Standard PCR was performed in 25-μl reactions, using Accuprime GC-rich DNA polymerase (Invitrogen) with the following reaction conditions: 95 °C for 3 min; 35 cycles of 95 °C for 30 s, 65 °C for 30 s and 72 °C for 1 min; and a 72 °C for 10 min extension with cooling to 4 °C. All PCR amplicons were verified on a 2% E-gel (Invitrogen) to ensure single amplified product. Transcriptome sequencing For library construction, 2–5 μg of total RNA was extracted from tumour samples by using Qiagen RNeasy Mini kits according to the manufacturer’s instructions. RNA concentration was measured by using a NanoDrop 100 Spectrophotometer (Thermo Scientific). RNA integrity was measured by using an Agilent Technologies 2100 Bioanalyzer Lab-on-a-chip system. Total RNA was treated with DNAse I (Invitrogen) and enriched for poly A-containing mRNA using oligo dT beads (Dynabeads, Invitrogen). The cDNA synthesis used random hexamers and the Superscript Double-Stranded cDNA Synthesis kit (Invitrogen). Paired-end reads from mRNA-seq were aligned to the following four database files by using a Burrows-Wheeler Aligner (0.5.5; (ref. 45 : (i) human NCBI Build 37 reference sequence, (ii) RefSeq, (iii) a sequence file representing all possible combinations of nonsequential pairs in RefSeq exons and (iv) AceView database flat file downloaded from UCSC, representing transcripts constructed from human expressed sequence tag (EST). The mapping results from databases (ii)–(iv) were aligned to human reference genome coordinates. The final BAM file (compressed binary version of the Sequence Alignment/Map format) file was constructed by selecting the best alignment in the four databases. The RNA expression level was measured by fragments per kilobase of transcript per million fragments mapped [46] . SVs were detected by using the CIRCERO algorithm, a novel algorithm that uses de novo assembly to identify SV in RNA-seq data (unpublished data). The structural variants detected in RNA-seq data were validated with MiSeq sequencing. Primer pairs were designed (with Primer3) to bracket the genomic regions containing putative SVs. The SVs found by RNA-seq are reported in Supplementary Table 4 . GISTIC analysis We used cghMCR (an R implementation of a modified version of the GISTIC analysis [47] ) to find regions that contained copy number alterations. We identified significantly amplified genes as those with segments of gain or loss (SGOL) scores 3 s.d.’s above the mean SGOL scores of all ‘gains’. Genes with SGOL scores 3 s.d.’s below the mean SGOL scores of all ‘losses’ were selected as significantly deleted genes. Timing of cn-LOH The cn-LOH regions were estimated from the CNA and LOH analysis data. When cn-LOH was identified in a pure tumour cell population, heterozygous alleles had become homozygous for either the reference allele or the alternative allele. Consequently, the MAF for SNVs accumulating before cn-LOH was either 0 (homozygous reference allele) or 1 (homozygous alternative allele), while SNVs occurring after cn-LOH had a maximum MAF of 0.5 (assuming no second mutation at the same locus) in tumour cells. We inferred the temporal order of cn-LOH and SNV accumulation in a genomic segment by comparing the AI values with the region’s MAF. Telomeric DNA content and telomere FISH The WGS data were analysed for total telomeric DNA content in tumours and matched germline DNA in 19 cases. Telomeric content reads containing (TTAGGG)4 or (CCCTAA)4 were counted and normalized to the average genomic coverage, and the log2 ratio of diagnostic and germline telomeric content estimates was then calculated to allow classification of telomeric content as gain, no change or loss [48] . Telomere FISH was performed on available formalin-fixed, paraffin-embedded tissue samples ( n =22) from the WGS and WES cohorts. Interphase FISH was performed on 4-μm-thick, formalin-fixed, paraffin-embedded tissue sections. The Cy3-labelled TelG probe (PNAbio) was co-denatured with the target cells on a hotplate at 90 °C for 12 min. The slides were incubated for 48 h at 37 °C and then washed in 4 M urea/2 × SSC at 45 °C for 5 min. Nuclei were counterstained with 200 ng ml −1 of 4′,6-diamidino-2-phenylindole (Vector Laboratories). The telomeric probe (red) hybridizes to telomeres on all chromosomes; a probe for 4p (green) was used as control. Analysis of microsatellite markers on chromosome 11p To identify commonly deleted regions on chromosome 11p15, we assessed LOH in 16 paired normal and tumour DNAs selected from the recurrence groups (WES) and in 22 additional IPACTR cases. We included peripheral blood DNA from 23 pairs of parents. Genomic DNA was extracted by using standard protocols. Fluorescence PCR semi-automated genotyping was used to detect and analyse allelic losses by using a panel of five microsatellite markers (D11S1363, D11S922, D11S4046, HUMTH01 and D11S988). TP53 and CTNNB1 mutations To detect and validate TP53 and CTNNB1 mutations, genomic DNA from ACT samples was tested by PCR-based bidirectional DNA sequencing of exons 2–11 and intron–exon boundaries for TP53 and exon 3 (codons 5–70) for CTNNB1 . Sequencing reactions were carried out on a high-throughput 3730xl DNA Analyzer (Applied Biosystems). TERT core promoter mutational status The TERT core promoter (HG19 coordinates, chr5: 1295151–1295347) was amplified in 19 paediatric ACT using PCR. Briefly, 10–20 ng of sample DNA was added to a 25-μl reaction containing amplitaq gold 360 master mix (Applied Biosystems) with 400 nM each of amplification primers (5′- CAGCGCTGCCTGAAACTCG -3′ (sense) and 5′- CCACGTGGCGGAGGGACT -3′ (antisense)) resulting in a PCR product of 197 bp. Sequencing reactions were carried out on a high-throughput 3730xl DNA Analyzer (Applied Biosystems). HHV6 chromosomal integration We amplified the sequences of the HHV6 major capsid protein and U94 genes in tumour and blood DNA from cases in the WGS and WES cohorts ( n =37). PCR and cycling conditions followed a previously described protocol [49] , [50] . Cases positive by PCR were tested using the FISH analysis. Peripheral blood mononuclear cells were cultured for 72 h in RPMI 1640 containing 20% FCS and 10 μg ml −1 phytohemagglutinin (PHA). After 1.0 h of colcemide treatment, cells were harvested according to the standard cytogenetic techniques. Cells in the metaphase were examined with FISH using HHV6 cosmid probes labelled by nick translation with fluorescein-dUTP and a dual-colour probe mapped to the sequences 5′ and 3′ of the common breakpoint region within the MLL locus (11q23; Abbott Molecular). The HHV6/ MLL probe mixture was applied to target metaphases and incubated at 37 °C overnight. After the slide was washed with 2 × SSC, 10 μl of 4,6-diamidino-2-phenylindole counterstain was applied to the target area for visualization. Accession codes. All whole-genome sequencing, whole-exome sequencing and transcriptome data have been deposited in the European Genome-phenome Archive (EGA), which is hosted by the European Bioinformatics Institute (EBI), under accession code EGAS00001000192. How to cite this article: Pinto, E. M. et al . Genomic landscape of paediatric adrenocortical tumours. Nat. Commun. 6:6302 doi: 10.1038/ncomms7302 (2015).